DOCK8 regulates protective immunity by controlling the function and survival of RORγt+ILCs Retinoic acid receptor-related orphan receptor-γt-positive (RORγt + ) innate lymphoid cells (ILCs) produce interleukin (IL)-22 and IL-17, which are critical for protective immunity against enteric pathogens. The molecular mechanism underlying the development and survival of RORγt + ILCs is not thoroughly understood. Here, we show that Dedicator of cytokinesis 8 (DOCK8), a scaffolding protein involved in cytoskeletal rearrangement and cell migration, is essential for the protective immunity against Citrobacter rodentium . A comparative RNA sequencing-based analysis reveals an impaired induction of antimicrobial peptides in the colon of DOCK8-deficient mice, which correlates with high susceptibility to infection and a very low number of IL-22-producing RORγt + ILCs in their GI tract. Furthermore, DOCK8-deficient RORγt + ILCs are less responsive to IL-7 mediated signalling, more prone to apoptosis and produce less IL-22 due to a defect in IL-23-mediated STAT3 phosphorylation. Our studies reveal an unsuspected role of DOCK8 for the function, generation and survival of RORγt + ILCs. The mammalian gastrointestinal (GI) tract harbours a large number of microbiota [1] . The mucosa of the GI tract is a critical interface for the host immune system and its associated microbial ecosystem [2] . At the barrier surfaces, innate lymphoid cells (ILCs) constitute a major fraction of the immune cell repertoire and serve a protective role in innate immune response to infectious microorganisms and in tissue remodelling after damage inflicted by injury or infection. ILCs are lineage-negative, Id2-dependent cells with varying functions [3] , [4] , [5] . Similar to T-helper cell lineage, ILCs are classified into three groups [6] , [7] based on their requirement of transcription factors and the effector cytokine production. Type 1 ILCs require transcription factor T-bet and produce interferon-γ, while type 2 ILCs (ILC2) depend on transcription factor GATA3 and produce Th2-associated cytokines interleukin-5 (IL)-5 and IL-13 (refs 5 , 6 ). Type 3 ILCs (ILC3) express RORγt transcription factor and produce IL-22 and/or IL-17 (refs 3 , 5 , 7 ). ILC3 include lymphoid tissue inducer cells (LTi) that mediate lymphoid tissue development in the fetus and its regeneration in the adult. Accordingly, RORγt-deficient mice lack LTi and lymph node (LN) formation [8] . Although the transcription factors important for the generation of these cells have been identified, little is known about the factors important for their maintenance and regulation of cytokine production. RORγt + ILCs produce large quantities of IL-22 (refs 9 , 10 , 11 , 12 , 13 , 14 ). IL-22 has been shown to promote wound healing, proliferation and antiapoptotic pathways in the intestinal epithelial cells [15] ; it also upregulates antimicrobial peptides and mucus production [9] , [16] . IL-22-mediated early induction of antimicrobial peptides, RegIIIγ and RegIIIβ in colonic epithelial cells is required for protection from Citrobacter rodentium ( C. rodentium ) infection [12] , [16] . Accordingly, IL-22-deficient mice show increased morbidity and mortality after C. rodentium infection [16] . The production of IL-22 by ILCs in response to C. rodentium infection is promoted by IL-23 (refs 12 , 16 , 17 ). Dedicator of cytokinesis 8 (DOCK8) interacts with the Rho family small G protein Cdc42 (refs 18 , 19 ). A very recent study has shown that in B cells, after ligation of TLR9, DOCK8 serves as an adaptor protein and links TLR9 to a STAT3 cascade, which is essential for TLR9-driven B-cell proliferation and differentiation [20] . DOCK8 mutation (null) is associated with combined immunodeficiency in humans [21] , [22] . DOCK8-deficient patients develop atopic dermatitis, Staphylococcus aureus skin abscesses or soft tissue infection, pneumonias, elevated serum IgE, eosinophilia and are more susceptible to cancer [21] , [23] . The majority of these patients have low numbers of CD4 + and CD8 + T cells in the blood and spleen [21] . However, it has not been investigated whether DOCK8-deficient patients also have defects in ILCs or altered microbial composition in their GI tracts, which would render them more susceptible to infections. Herein, we present evidence that DOCK8 is essential for protective immunity against an enteric pathogen. Using DOCK8-deficient mice, we have shown that DOCK8 plays a crucial role in the survival of RORγt + ILCs and their cytokine production. Indeed, we further determined that RORγt + ILCs require DOCK8 for optimal STAT3 activation and IL-22 production on IL-23 stimulation. Therefore, our studies suggest that besides having defective B-cell-mediated responses, DOCK8-deficient patients may also have limited numbers of ILC3. Thus, our studies may help explain why the absence of DOCK8 contributes to patients’ susceptibility to a broad spectrum of pathogens. DOCK8 is required for the clearance of an enteric pathogen To define the role of scaffolding protein DOCK8 in IL-23-mediated induction of IL-22, we utilized DOCK8 pri/pri mice [24] . These mice had defects in B-cell immunological synapses, germinal centre formation and long-lived antibody production. Along with B-cell defects, these mice also had a defect in T-cell survival and function [25] . Therefore, we first examined the total cell number as well as the cell composition in DOCK8 pri/pri mice. As previously shown, these mice have significantly fewer cells in spleen and LNs in comparison with age and sex-matched wild-type (WT) mice ( Supplementary Fig. 1a , top). In contrast to the peripheral cell count, DOCK8 pri/pri mice have a comparable number of lamina propria lymphocytes (LPL) in the GI tract, but significantly higher cells in the mesenteric LN in comparison with WT mice ( Supplementary Fig. 1a , bottom). Consistent with previous findings, CD4 + and CD8 + T cells in the spleens of DOCK8 pri/pri mice were reduced by 50–60% of WT levels [25] , [26] . In addition, we did not find significant changes in the numbers of CD4 + and CD8 + T cells in the lamina propria (LP) of DOCK8 pri/pri mice in comparison with WT ( Supplementary Fig. 1b ). Interestingly, DOCK8 deficiency did not affect the number of mature B cells in lymphoid organs except in the small intestine (SI), where we found a significant reduction of the B-cell percentage ( Supplementary Fig. 1c ). This reduction was also more pronounced when mice were infected with C. rodentium ( Supplementary Figs 1d and 2 ). The B cells that were found in the colonic LP expressed high levels of major histocompatibility complex (MHC) Class II ( Supplementary Fig. 1d ). DOCK8 has been shown to be critical for interstitial dendritic cell (DC) migration during immune responses [26] . Therefore, we assessed whether DOCK8 deficiency could affect the recruitment of myeloid cells in response to an infection. However, we did not find any reduction in the recruitment of CD11b + or CD11c + cells to the LP of DOCK8 pri/pri mice after infection with C. rodentium ( Supplementary Fig. 1e ). Since it has been shown that B cells play an important role in the clearance of enteric pathogens [27] , [28] , [29] , we infected WT, DOCK8 pri/pri mice, B-cell-deficient (μMT) and IL-23 R −/− mice with C . rodentium. Interestingly, similar to IL-23R −/− mice, all DOCK8 pri/pri mice lost weight and succumbed to the infection ( Fig. 1a,b ). The spleens and livers of DOCK8 pri/pri mice contained two to four log more bacteria than WT, indicating that DOCK8 pri/pri mice were unable to control bacterial dissemination ( Fig. 1c ). Although we observed a defect in the recruitment of MHC class II high B cells to the GI tract of DOCK8 pri/pri mice ( Supplementary Figs 1c,d and 2 ), μMT mice survived and were able to clear the infection ( Fig. 1a,b ). These results suggest that DOCK8 deficiency renders mice susceptible to C. rodentium infection independently of B cell function. IL-22 −/− and IL-23p19 −/− mice are highly susceptible to C. rodentium infection [16] , [30] , [31] . Therefore, we used IL-23R −/− mice as a positive control for infection. Consistent with above, IL-23R −/− mice were highly susceptible to infection ( Fig. 1a,b ). 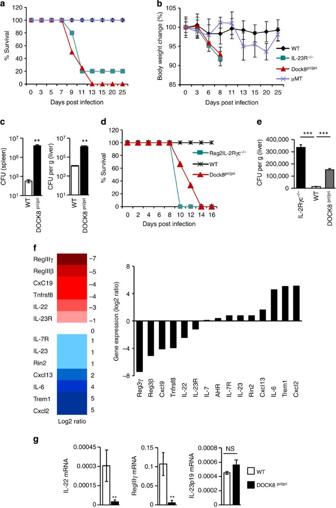Figure 1: DOCK8 is required for the clearance of enteric pathogen. (a–c) WT, IL-23R−/−, DOCK8pri/priand μMT mice were infected withC. rodentium(a) percent survival and (b) average body weight change of WT (n=5), IL-23R−/−(n=5), DOCK8pri/pri(n=6) and μMT (n=4) mice after infection. (c)C. rodentiumcolony-forming units (CFU) in the spleens and livers of infected mice at day 8 post infection (p.i.). (d,e) DOCK8 is required in haematopoietic compartment for the survival. Bone marrow cells from mice of indicated genotype were transferred into irradiated Rag2−/−IL-2 Rγc−/−mice. (d) Percent survival and (e)C. rodentiumCFU in the livers of infected mice at day 8 p.i. (f) DOCK8-dependent gene expression in the colons ofC. rodentiuminfected mice. (g) ColonicIL-22,RegIIIγ andIL-23p19expression in response to infection at day 8 p.i. Three independent experiments were performed with a minimum of four to six mice per group. The data shown are the mean±s.d.Pvalues were obtained by Student’st-test. **P<0.01, ***P<0.001. NS, not significant. Figure 1: DOCK8 is required for the clearance of enteric pathogen. ( a – c ) WT, IL-23R −/− , DOCK8 pri/pri and μMT mice were infected with C. rodentium ( a ) percent survival and ( b ) average body weight change of WT ( n =5), IL-23R −/− ( n =5), DOCK8 pri/pri ( n =6) and μMT ( n =4) mice after infection. ( c ) C. rodentium colony-forming units (CFU) in the spleens and livers of infected mice at day 8 post infection (p.i.). ( d , e ) DOCK8 is required in haematopoietic compartment for the survival. Bone marrow cells from mice of indicated genotype were transferred into irradiated Rag2 −/− IL-2 Rγc −/− mice. ( d ) Percent survival and ( e ) C. rodentium CFU in the livers of infected mice at day 8 p.i. ( f ) DOCK8-dependent gene expression in the colons of C. rodentium infected mice. ( g ) Colonic IL-22 , RegIII γ and IL-23p19 expression in response to infection at day 8 p.i. Three independent experiments were performed with a minimum of four to six mice per group. The data shown are the mean±s.d. P values were obtained by Student’s t -test. ** P <0.01, *** P <0.001. NS, not significant. Full size image Next, we determined whether DOCK8 was required within haematopoietic cells or non-haematopoietic cells. We generated chimeras by transferring bone marrow cells isolated from either DOCK8 pri/pri or WT littermate mice into irradiated Rag2 −/− IL-2Rγ −/− mice. Five weeks after transfer, these mice were infected with C. rodentium . As expected, similar to Rag2 −/− IL-2Rγ −/− mice, all Rag2 −/− IL-2Rγ −/− mice transferred with DOCK8 pri/pri bone marrow succumbed to the infection, while WT bone marrow transferred mice survived the infection ( Fig. 1d ). The livers of Rag2 −/− IL-2Rγ −/− mice and Rag2 −/− IL-2Rγ −/− mice transferred with DOCK8 pri/pri bone marrow contained significantly higher bacterial load than those transferred with WT bone marrow cells ( Fig. 1e ). These results suggest that DOCK8 is required within the haematopoietic compartment and plays an important role in the function of immune cells involved in protective immunity. To understand the effect of DOCK8 on global transcription levels, we used RNA sequencing to examine the differential gene expression on C. rodentium infection. RNA was purified from the infected colons of WT and DOCK8 pri/pri mice. We evaluated the levels of the gene expression in the infected colons of WT and DOCK8 pri/pri mice. Among the most highly expressed genes, RegIII γ, RegIII β and IL-22 were highly defective in DOCK8 pri/pri mice, in comparison with WT mice ( Fig. 1f ). Since it has been shown that early IL-22-dependent induction of RegIIIγ is critical for protective immunity against enteric pathogen [12] , [16] , we measured colonic IL-22 and RegIII γ transcripts after infection with C. rodentium . Consistent with RNA-seq data, the levels of IL-22 and RegIII γ expression were very low in the colon of DOCK8 pri/pri mice in comparison with levels found in the colon of WT mice ( Fig. 1g ). This finding indicates that DOCK8 is required for the induction of IL-22 expression on infection. IL-22 can be produced by many cell types, including ILCs and Th22 cells [3] , [9] , [11] , [12] , [31] , [32] , [33] . Therefore, we addressed the cellular source of IL-22 that was critical for protection against enteric pathogen infection. To assess whether DOCK8 is required for IL-22 production by ILCs or Th22, we crossed DOCK8 pri/pri mice with Rag1 −/− mice lacking T cells. These mice were also highly susceptible to enteric pathogen infection and failed to clear infection ( Supplementary Fig. 3a,b ). The spleens and livers of Rag1 −/− DOCK8 pri/pri mice contained significantly more bacteria than Rag1 −/− mice, indicating that DOCK8 is required in innate immune cells for the control of enteric pathogen infection ( Supplementary Fig. 3c ). And similar to DOCK8 pri/pri mice, Rag1 −/− DOCK8 pri/pri mice were also highly defective in IL-22 -dependent RegIII γ induction after enteric pathogen infection ( Supplementary Fig. 3d ). All together, these data indicate that DOCK8 is required for protective immunity against C. rodentium by regulating IL-22 production from innate immune cells. Exogenous IL-22 protects DOCK8 KO mice during C. rodentium infection Our data ( Fig. 1 and Supplementary Fig. 3 ) clearly showed that DOCK8 was required for controlling C. rodentium infection. To test whether exogenous IL-22 could rescue the DOCK8 pri/pri mice on C. rodentium infection, we injected IL-22 cDNA via hydrodynamic delivery into DOCK8 pri/pri mice. We had previously shown that a single injection of IL-22-encoding cDNA into IL-22-defective mice restored expression of IL-22 in the blood and colon, lasted as long as 10 days [34] . We gave one injection of IL-22-encoding plasmid 2 days before infection and another at day 5 post infection. DOCK8 pri/pri mice that received the IL-22 plasmid survived an average of 5 days longer and had significantly less weight loss compared to empty plasmid recipients ( Fig. 2a,b ). In the IL-22 plasmid-treated group, splenic and liver bacteria counts were significantly lower compared to the empty plasmid-injected group ( Fig. 2c ). Thus, these sets of experiments collectively demonstrated that defective IL-22 production was an important cause of high bacteria load and death of DOCK8 pri/pri mice during C. rodentium infection. Conversely, only 15% of DOCK8 pri/pri mice that received the IL-22 plasmid survived the infection, suggesting that these mice might have other defects in innate immune cells, which were required for further survival. DOCK8 has been shown to be important for B-cell immunological synapses, germinal centres and long-lived antibody production [24] . It is also important for the survival and function of CD8 + T and NKT cells [25] , [35] . The DOCK8 deficiency also results in reduced CD4 + T cells and defective interstitial DC migration during immune responses [25] , [26] . These previous findings suggest that DOCK8 is also required for fully functional acquired immune response. It is important to mention that mice defective in the recombination activating gene become predisposed to C. rodentium infection at 3 to 4 weeks post infection, suggesting that both innate and acquired immune response is required to clear C. rodentium infection ( Supplementary Fig. 3a,b ) [12] , [16] . Thus, partial restoration of survival in DOCK8 pri/pri mice injected with IL-22 plasmid could be due to defective acquired immune responses. 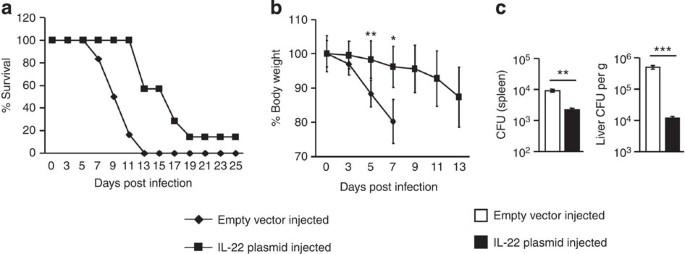Figure 2: Exogenous IL-22 protects DOCK8 KO mice duringC. rodentiuminfection. DOCK8pri/primice were administered with IL-22 expressing plasmid or empty vector via hydrodynamic injections at −2 and +5 days ofC. rodentiuminfection. (a) Percent survival (b) average body weight changes after infection and (c) colony-forming units in the spleens and livers of infected mice. All the data are representative of three independent experiments with five mice per group. The data shown are the mean±s.d.Pvalues were obtained by Student’st-test. *P<0.05, **P<0.01, ***P<0.001. Figure 2: Exogenous IL-22 protects DOCK8 KO mice during C. rodentium infection. DOCK8 pri/pri mice were administered with IL-22 expressing plasmid or empty vector via hydrodynamic injections at −2 and +5 days of C. rodentium infection. ( a ) Percent survival ( b ) average body weight changes after infection and ( c ) colony-forming units in the spleens and livers of infected mice. All the data are representative of three independent experiments with five mice per group. The data shown are the mean±s.d. P values were obtained by Student’s t -test. * P <0.05, ** P <0.01, *** P <0.001. Full size image RORγt + ILCs require DOCK8 for optimal IL-22 production Prior reports undoubtedly showed that ILC3 plays a decisive role in protection against C. rodentium infection by producing IL-22 early on [9] , [10] , [12] , [13] , [36] , [37] , [38] . In this model, early during infection, classical DCs produce IL-23 that induces IL-22 production via ILC3 (refs 12 , 16 , 17 ). IL-22 enhances epithelial cell repair and prevents dissemination of bacteria. Therefore, we analysed whether the defect in IL-22 production by DOCK8-deficient ILCs resulted from direct DOCK8-mediated signalling in ILCs or resulted from an indirect effect of DOCK8 on other cells important for its function. The defective IL-22 production in DOCK8 pri/pri mice could be due to defective IL-23 expression in DCs. Therefore, we measured IL-23p19 , a specific subunit of IL-23, in the colon of C. rodentium infected mice. Interestingly, IL-23 expression in the colon of C. rodentium infected DOCK8 pri/pri mice was comparable to that of WT mice ( Fig. 1g ), suggesting that the IL-22 defect in DOCK8 pri/pri mice is not due to the impaired IL-23 expression in DCs. We also analysed the expression of Dock8 in innate IL-23R + cells and have found that Dock8 was highly expressed in these cells ( Supplementary Fig. 4 ). Next we investigated whether DOCK8 was also required for IL-22 production by RORγt + ILCs on IL-23 stimulation. Therefore, we examined IL-22 expression in the LPLs isolated from DOCK8 pri/pri mice and their littermate control WT mice. As expected, in WT mice, ILC3 (CD3 negative) produced high amounts of IL-22 in response to IL-23. Compared with those in WT mice, both the percentage and absolute number of CD3 − IL-22 + cells in the GI tract of DOCK8 pri/pri mice were significantly reduced, indicating that DOCK8 was important for the production of IL-22 in the GI tract ( Fig. 3a,b ). However, this result could be misleading due to the paucity of RORγt + ILC3 in DOCK8 pri/pri mice that could have led to an overall reduction of IL-22 production. Thus, it remains uncertain whether DOCK8 directly regulates IL-22 production from each individual ILC3. To verify this, we purified CD90.2 + IL-23R + cells from the SI LPLs of Rag1 −/− IL-23R gfp/+ or Rag1 −/− IL-23R gfp/+ DOCK8 pri/pri mice and cultured them with or without IL-23. The IL-22 protein in the culture supernatant was measured by enzyme-linked immunosorbent assay (ELISA). The production of IL-22 by DOCK8-deficient RORγt + ILCs was significantly reduced compared with those in WT mice ( Fig. 3c ). To further corroborate our findings, we measured IL-22 and IL-17 transcript levels in sorted ILC3s from Rag1 −/− IL-23R gfp/+ or Rag1 −/− IL-23R gfp/+ DOCK8 pri/pri mice ( Supplementary Fig. 5 ). The IL-22 transcript level in DOCK8-deficient ILC3s was significantly reduced compared to those in WT mice. However, IL-17A transcript level was comparable in WT and DOCK8-deficient ILC3s. These results suggested that DOCK8 was required for RORγt + ILCs optimal IL-22 production in response to IL-23 stimulation. We also investigated the function of DOCK8 on IL-22 production by CD4 + T cells after C. rodentium infection. DOCK8-deficient CD4 + T cells are highly defective in IL-22 production after C. rodentium infection ( Supplementary Fig. 6 ). However, IL-22 produced by CD4 + T cells for protection against C. rodentium is not as crucial as IL22 produced by ILC3 (ref. 39 ). Since IL-23 signals via STAT3-dependent mechanisms, we tested whether DOCK8 was also required in ILC3 for the activation of STAT3 in response to IL-23 stimulation. Thus, we stimulated freshly isolated ILC3 with IL-23 and assessed STAT3 phosphorylation (pY 705 -STAT3) by flow cytometry ( Fig. 3d ). Consistent with the IL-23-mediated STAT3 phosphorylation in T cells [40] , IL-23 induced STAT3 phosphorylation in WT ILCs; however, IL-23-mediated STAT3 activation was severely impaired in DOCK8-deficient ILCs ( Fig. 3d ). This data clearly show that DOCK8 is required for STAT3 activation and IL-22 production on IL-23 stimulation. 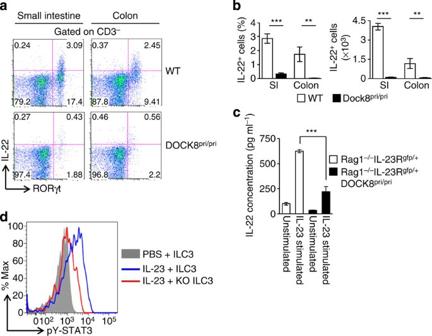Figure 3: DOCK8 is also required for the IL-23-mediated induction of IL-22. (a) SI LPLs from WT and DOCK8pri/primice were stimulated with 20 ng ml−1IL-23 for 4 h in the presence of Golgi stop. RORγt and IL-22 expression in CD3−cells was analysed by flow cytometry. (b) Percentage and absolute numbers of intestinal CD3−IL-22+cells. (c) Sorted ILC3 (CD90.2+IL-23Rgfp/+) from intestinal LPLs of Rag1−/−IL-23Rgfp/+and Rag1−/−IL-23Rgfp/+DOCK8pri/primice were cultured with or without IL-23 (20 ng ml−1). The IL-22 produced in culture supernatant was measured by ELISA. (d) Fluorescence-activated cell sorting analysis for detection of pSTAT3 in ILC3 from Rag1−/−IL-23Rgfp/+or Rag1−/−IL-23Rgfp/+DOCK8pri/primice. All the data are representative of three independent experiments with three mice per group. The data shown are the mean±s.d.Pvalues were obtained by Student’st-test. **P<0.01, ***P<0.001. Figure 3: DOCK8 is also required for the IL-23-mediated induction of IL-22. ( a ) SI LPLs from WT and DOCK8 pri/pri mice were stimulated with 20 ng ml −1 IL-23 for 4 h in the presence of Golgi stop. RORγt and IL-22 expression in CD3 − cells was analysed by flow cytometry. ( b ) Percentage and absolute numbers of intestinal CD3 − IL-22 + cells. ( c ) Sorted ILC3 (CD90.2 + IL-23R gfp/+ ) from intestinal LPLs of Rag1 −/− IL-23R gfp/+ and Rag1 −/− IL-23R gfp/+ DOCK8 pri/pri mice were cultured with or without IL-23 (20 ng ml −1 ). The IL-22 produced in culture supernatant was measured by ELISA. ( d ) Fluorescence-activated cell sorting analysis for detection of pSTAT3 in ILC3 from Rag1 −/− IL-23R gfp/+ or Rag1 −/− IL-23R gfp/+ DOCK8 pri/pri mice. All the data are representative of three independent experiments with three mice per group. The data shown are the mean±s.d. P values were obtained by Student’s t -test. ** P <0.01, *** P <0.001. Full size image Profound reduction of RORγt + ILCs in the absence of DOCK8 The major innate cell population that expresses IL-23R in the intestine is group 3 ILC, which is composed of LTi cells and ILC3s [41] . Various ILC3s were described in humans and mice based on the effector cytokines they produce. These include but are not limited to (1) IL-22-producing NCR + ILC3 (ref. 9 ), which are also called ILC22, NK22, NKR-LTi or NCR22 (ref. 42 ) (2) NCR − IL-17A + IFN-γ + double producing ILC3 (ref. 43 ) and lastly (3) NCR − IL-17A + ILC3s [44] . All of these subsets of ILC3s respond to IL-23 and produce the above-mentioned cytokine. Thus, the group 3 of ILCs is very heterogeneous and is composed by numerous subsets of cells that can be distinguished by the expressions of various surface markers such a CD4 and NKp46. To determine whether DOCK8 deficiency affects the development of a particular subset of ILC3 in the GI tract, we examined the RORγt + ILC compartment of DOCK8 pri/pri mice. Thus, we stained both the SI and colon lamina propria leukocytes (LPLs) with CD3, CD90.2, CD127, RORγt, CD4 and NKp46-specific antibodies. Both the percentage and number of RORγt + ILCs (CD3 − CD90.2 + CD127 + RORγt + ) in the SI and colon were significantly reduced in DOCK8 pri/pri mice ( Fig. 4a–c and Supplementary Fig. 7a–c ). The number of RORγt + ILCs in the LPLs of SI of DOCK8 pri/pri mice was reduced to 5.6% of the number in WT mice. The percentage of CD4 + and NKp46 + ILCs among RORγt + ILCs was comparable between DOCK8 pri/pri and WT mice, despite the fact that their absolute numbers were significantly reduced in DOCK8 pri/pri mice ( Fig. 4a–c and Supplementary Fig. 7a–c ). Next, we investigated whether the defect of RORγt + ILCs in DOCK8 pri/pri mice was only limited to the gut, or could be observed also in other organs. Both the percentage and absolute numbers of RORγt + ILCs were significantly reduced in multiple organs of DOCK8-deficient mice, including spleens and LNs ( Supplementary Fig. 8a–c ). Thus, DOCK8 is not only important for the survival of RORγt + ILCs of the gut, but it is also required for their maintenance in other organs as well. We further explored whether DOCK8 requirement by RORγt + ILCs was perinatal or postnatal. Therefore, we assessed the number of RORγt + ILCs in the gut of WT and DOCK8 pri/pri newborn mice. In contrast to the significant decrease of RORγt + ILCs in the gut LPLs of adult DOCK8 pri/pri mice, the frequency of total RORγt + and perinatal CD4 + LTi cells in the gut LPLs isolated from DOCK8 pri/pri newborn mice was comparable to those from WT newborns, suggesting that DOCK8 is dispensable for the development of perinatal LTi cells in the gut ( Supplementary Fig. 9a–c ). Recently, it was shown that ILC3s could be identified as CD45 low and CD90.2 high cells [39] . Therefore, to sort perinatal LTi cells, we stained newborn mice GI tract LPLs with CD45, CD3, CD90.02 and RORγt and assessed whether CD3 − CD45 low and CD90.2 high cells could represent RORγt + cells, as in adult mice ( Supplementary Fig. 9d , upper panel). Consistent with recently published work [39] , most of the RORγt + cells found in LP of newborn mice could be identified as CD3 − CD45 low and CD90.2 high cells. Then, we sorted CD4 + and CD4 − perinatal LTi cells and assessed the expression of Dock8 . Our result showed that CD4 + LTi cells do express Dock8 transcripts, but that expression level was significantly reduced compared with CD4 − LTi and adult ILC3s ( Supplementary Fig. 9d,e ). All together, these results suggest that DOCK8 is dispensable for the development of perinatal LTi cells in the gut. 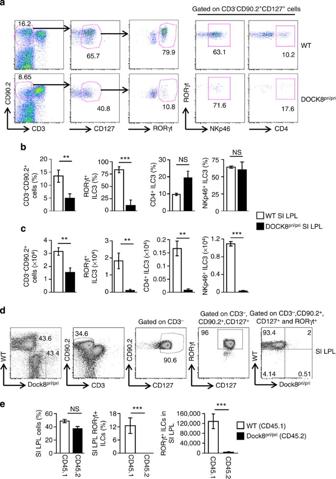Figure 4: Profound reduction of RORγt+ILCs in the absence of DOCK8. (a) RORγt+ILCs were analysed in SI LPLs by flow cytometry after gating on CD3−CD90.2+CD127+cells. (b,c) Percentage and absolute numbers of CD3−CD90.2+, CD3−CD90.2+CD127+RORγt+, CD3−CD90.2+CD127+RORγt+CD4+and CD3−CD90.2+CD127+RORγt+NKp46+cells of WT and DOCK8pri/primice. (d,e) Cell-intrinsic functions of DOCK8 regulate RORγt+ILCs. Mixed bone marrow chimeras generated by reconstituting 50% CD45.1 WT and 50% CD45.2 DOCK8pri/primice and transferred into lethally irradiated Rag2−/−IL-2Rγc−/−mice. (d) RORγt+ILCs (CD3−CD90.2+CD127+) were analysed 4 weeks post transfer. (e) The percentage and absolute number of RORγt+ILCs. Three independent experiments were performed with a minimum of three mice per group. The data shown are the mean±s.d.Pvalues were obtained by Student’st-test. **P<0.01, ***P<0.001. NS, not significant. Figure 4: Profound reduction of ROR γ t + ILCs in the absence of DOCK8. ( a ) RORγt + ILCs were analysed in SI LPLs by flow cytometry after gating on CD3 − CD90.2 + CD127 + cells. ( b , c ) Percentage and absolute numbers of CD3 − CD90.2 + , CD3 − CD90.2 + CD127 + RORγt + , CD3 − CD90.2 + CD127 + RORγt + CD4 + and CD3 − CD90.2 + CD127 + RORγt + NKp46 + cells of WT and DOCK8 pri/pri mice. ( d , e ) Cell-intrinsic functions of DOCK8 regulate RORγt + ILCs. Mixed bone marrow chimeras generated by reconstituting 50% CD45.1 WT and 50% CD45.2 DOCK8 pri/pri mice and transferred into lethally irradiated Rag2 −/− IL-2Rγc −/− mice. ( d ) RORγt + ILCs (CD3 − CD90.2 + CD127 + ) were analysed 4 weeks post transfer. ( e ) The percentage and absolute number of RORγt + ILCs. Three independent experiments were performed with a minimum of three mice per group. The data shown are the mean±s.d. P values were obtained by Student’s t -test. ** P <0.01, *** P <0.001. NS, not significant. Full size image To further confirm our findings, we crossed DOCK8 pri/pri mice with Rag1 −/− IL-23R gfp/+ and generated Rag1 −/− IL-23 gfp/+ DOCK8 pri/pri mice in which IL-23R expression can be followed based on GFP expression [45] . These mice have fewer CD90.2 + IL-23R + cells compared with littermate control mice ( Supplementary Fig. 10a ). We also measured the level of IL-23R transcripts in the colons of Rag1 −/− IL-23 gfp/+ DOCK8 pri/pri mice after C. rodentium infection. Consistent with DOCK8 pri/pri mice, these mice also had significantly fewer IL-23R transcripts in comparison with Rag1 −/− IL-23R gfp/+ mice ( Supplementary Fig. 10b,c ). Altogether, these results indicate that DOCK8 is involved in the development or survival of RORγt + IL-23R + ILCs. To determine whether DOCK8 was only required for the survival of RORγt + ILCs, we compared the effect of DOCK8 deficiency on the generation of ILC2 in the GI tract LPLs ( Supplementary Fig. 11a,b ). In contrast to ILC3 in the gut of DOCK8-deficient mice, ILC2 absolute numbers of DOCK8-deficient mice did not significant differ from the number of ILC2s found in DOCK8-sufficient mice. Interestingly, the percentage of ILC2 was inversely correlated with the percentage of ILC3 in DOCK8-deficient mice and was significantly elevated in DOCK8-deficient mice. These data suggest that DOCK8 deficiency specifically influences the generation/survival of RORγt + ILCs, but not GATA3 + ILC2, in the gut. To investigate whether the reduction in RORγt + ILCs is due to a cell-intrinsic defect, we generated mixed bone marrow chimeric mice in which 50% of the reconstituting bone marrow was derived from WT CD45.1 donors and 50% was derived from DOCK8 pri/pri CD45.2 congenic donors. Thus, WT and DOCK8 pri/pri cells could be distinguished on the basis of CD45.1 and CD45.2 expressions, respectively. We then evaluated the generation of RORγt + ILCs in these chimeric mice. DOCK8-deficient haematopoietic progenitor cells failed to give rise to RORγt + ILCs, whereas WT bone marrow progenitors developed normally into RORγt + ILCs in irradiated Rag2 −/− IL-2Rγ −/− mice ( Fig. 4d,e and Supplementary Fig. 7d,e ). These data suggest an intrinsic requirement of DOCK8 for the development of RORγt + ILCs. Our data clearly show that DOCK8 is required for the generation/survival/function of ILC3. To test whether the infusion of WT ILC3 could provide innate immune protection on C. rodentium infection, 5 × 10 3 ILC3 sorted from Rag1 −/− IL-23R gfp/+ host was adaptively transferred in to Rag1 −/− DOCK8 pri/pri mice 1 h after infection. DOCK8 pri/pri mice that received the ILC3 survived an average of 3.5 days longer and had significantly less weight loss compared with untreated recipients ( Supplementary Fig. 12a,b ). In the ILC3-transfered group, splenic and liver bacteria counts were significantly lower compared with the untreated group ( Supplementary Fig. 12c ). Interestingly, the mean survival of DOCK8-deficient mice infused with WT ILC3s is comparable to the mean survival observed in mice that lack function ILC3s that were infused with WT ILC3s [12] , [39] . It remains unclear why the adoptive transfer of WT ILCs could only provide partial protection, one possible explanation is that only limited number of transferred ILC3s can migrate to the colon or these cells have a short life span. In a recent study, DOCK8 was shown to interact with Myd88 in B cells [20] . However, we found that Myd88 was dispensable for the generation of RORγt + ILCs ( Supplementary Fig. 13 ). This result is consistent with prior findings, in which Myd88 −/− mice did not show significant alteration in the development of RORγt + ILCs [46] . DOCK8 also interacts with WASp and regulates natural killer cell cytotoxicity [47] . However, we did not find significant reductions of RORγt + ILC3 in WASp −/− mice ( Supplementary Fig. 13 ). Thus, DOCK8 is required for RORγt + ILCs development in a cell-intrinsic manner and independent of Myd88 or WASp-mediated functions. Generation and survival of RORγt + ILCs requires DOCK8 To address why DOCK8 pri/pri mice have drastic reductions in RORγt + ILCs, we first tested whether these mice had an intact common lymphoid progenitors (CLPs) compartment. RORγt + ILCs develop from CLPs (Lin − Sca-1 low c-Kit Int IL-7Rα + ) [48] , [49] ; thus, we evaluated the number of these cells in the bone marrow of WT and DOCK8 pri/pri mice ( Fig. 5a ). Interestingly, we did not find any major difference in the percentage of CLPs among WT or DOCK8 pri/pri mice. These data are consistent with the fact that DOCK8-deficient mice have normal LNs and DOCK8 may be required for RORγt + ILCs survival only after birth. Next, we assessed whether DOCK8-deficient RORγt + ILCs had a developmental defect due to defects in transcription factors implicated in their generation. These cells require transcription factors Id2 (refs 4 , 50 ), RORγt [51] and Tox [52] for their development. Previous work in our laboratory has clearly shown all CD90.2 + IL-23R + cells are RORγt + ILCs [34] . Therefore, we purified CD90.2 + IL-23R + and CD90.2 + IL-23R − cells from Rag1 −/− IL-23R gfp/+ DOCK8 pri/pri and Rag1 −/− IL-23R gfp/+ mice and measured transcripts for Id2 , Tox and ROR γ t by quantitative PCR. However, we observed comparable expression of these transcription factors in CD90.2 + IL-23R + cells purified from the GI tract of Rag1 −/− IL-23R gfp/+ DOCK8 pri/pri mice in comparison to controls ( Supplementary Fig. 14 ). These data further support the idea that DOCK8 is not required for early development of RORγt + ILCs, but may be required for their maintenance or survival. Recently, the aryl hydrocarbon receptor (Ahr), a ligand-dependent transcription factor, was shown to be important for the generation and maintenance of adult RORγt + ILCs [10] , [37] , [38] . Therefore, we also examined Ahr transcripts by quantitative PCR, but its level of expression in CD90.2 + IL-23R + cells was comparable to the levels found in WT cells ( Supplementary Fig. 14 ). These data indicate that the effect of DOCK8 on RORγt + ILCs occurs independently of Ahr expression. Recently, it has been shown that Notch signalling is necessary for adult, but not fetal, development of RORγt + ILCs [48] . Thus, we examined the expression of Notch-1 and Notch-2 transcript in CD90.2 + IL-23R + cells from Rag1 −/− IL-23R gfp/+ and Rag1 −/− IL-23R gfp/+ DOCK8 pri/pri mice. CD90.2 + IL-23R + cells from Rag1 −/− IL-23R gfp/+ DOCK8 pri/pri mice had comparable expression of Notch-2 , but slightly higher expression of Notch-1 ( Supplementary Fig. 15 ). We also assessed the transcript of Hes1 , a Notch transcriptional target, in CD90.2 + IL-23R + cells but its expression was comparable. However, CD90.2 + IL-23R − cells from Rag1 −/− IL-23R gfp/+ DOCK8 pri/pri mice had significantly higher expression of Hes1 transcript ( Supplementary Fig. 15 , top panel). More importantly, we transduced bone morrow haematopoietic stem cells (HSCs) of DOCK8-deficient mice with retrovirus that contained constitutively active intracellular Notch and infused the transduced HSCs into Rag1IL2Rγ-deficient mice recipient. Three weeks after HSC reconstitution, we analysed the number of ILC3 in the gut of these transduced HSC-reconstituted mice. In these mice, the number of ILC3 was vey limited. Thus, the overexpression of intracellular Notch could not rescue the ILC3 compartment in the absence of DOCK8 ( Supplementary Fig. 15 , bottom panel). Therefore, it is very unlikely that ILC3s defects observed in DOCK8-deficient mice are due to a defect in Notch mediated functions. 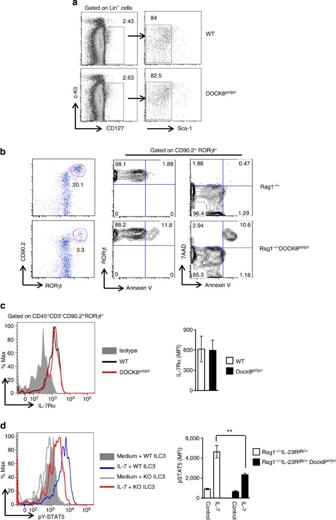Figure 5: DOCK8 is required for the generation and survival of RORγt+ILCs. (a) Dot plots showing the bone marrow CLPs from WT and DOCK8pri/primice. (b) DOCK8-deficient RORγt+ILC3s have enhanced apoptosis. Rag1−/−and Rag1−/−DOCK8pri/priSI LPLs were examined by flow cytometry for RORγt and apoptosis markers (Annexin V and 7-AAD). All the data are representative of three independent experiments with three mice per group. (c) Histogram showing the IL-7Rα expression on ILC3 (left panel) and bar graph showing the MFI of IL-7Rα expression (right panel) (d) Histogram showing the phosphorylation of STAT5 in ILC3 on IL-7 stimulation (left panel) and bar graph showing the MFI of pSTAT5 in ILC3 isolated from the SI LPLs of Rag1−/−IL-23Rgfp/+or Rag1−/−IL-23Rgfp/+DOCK8pri/primice (right panel). All the data are representative of four independent experiments with two to four mice per group. The data shown are the mean±s.d.Pvalues were obtained by Student’st-test. **P<0.01. Figure 5: DOCK8 is required for the generation and survival of ROR γ t + ILCs. ( a ) Dot plots showing the bone marrow CLPs from WT and DOCK8 pri/pri mice. ( b ) DOCK8-deficient RORγt + ILC3s have enhanced apoptosis. Rag1 −/− and Rag1 −/− DOCK8 pri/pri SI LPLs were examined by flow cytometry for RORγt and apoptosis markers (Annexin V and 7-AAD). All the data are representative of three independent experiments with three mice per group. ( c ) Histogram showing the IL-7Rα expression on ILC3 (left panel) and bar graph showing the MFI of IL-7Rα expression (right panel) ( d ) Histogram showing the phosphorylation of STAT5 in ILC3 on IL-7 stimulation (left panel) and bar graph showing the MFI of pSTAT5 in ILC3 isolated from the SI LPLs of Rag1 −/− IL-23R gfp/+ or Rag1 −/− IL-23R gfp/+ DOCK8 pri/pri mice (right panel). All the data are representative of four independent experiments with two to four mice per group. The data shown are the mean±s.d. P values were obtained by Student’s t -test. ** P <0.01. Full size image DOCK8 has been implicated in the survival and function of CD8 + T cells and NKT cells [25] , [35] . Therefore, we next investigated if DOCK8 also influences the survival of RORγt + ILCs in the GI tract. We stained SI LPLs with 7-AAD and Annexin V to examine the apoptotic cell death. In contrast to CD90.2 + RORγt + cells in the GI tract of Rag1 −/− mice, CD90.2 + RORγt + cells isolated from Rag1 −/− DOCK8 pri/pri mice consistently showed higher Annexin V and 7-AAD staining ( Fig. 5b ), indicating that intestinal RORγt + ILCs without DOCK8 are more prone to apoptosis. However, the expression of antiapoptotic gene Bcl-2 was not affected in DOCK8 pri/pri mice ILCs, as shown by fluorescence-activated cell sorting histogram ( Supplementary Fig. 16a ). Next, we analysed the expression of antiapoptotic genes, Bcl-2 , Bcl-xL and Mcl-1 in CD90.2 + IL-23R + cells from Rag1 −/− IL-23R gfp/+ and Rag1 −/− IL-23R gfp/+ DOCK8 pri/pri mice. CD90.2 + IL-23R + cells from Rag1 −/− IL-23R gfp/+ DOCK8 pri/pri mice had lower expression of Bcl-xL but no significant difference in expressions of Bcl-2 or Mcl-1 ( Supplementary Fig. 16b ). Thus, DOCK8 may promote the survival of RORγt + ILCs by inducing Bcl-xL expression. Since the survival and the generation of RORγt + ILCs are largely dependent on IL-7 (refs 53 , 54 ) mediated signalling, we analysed the IL-7Rα expression on RORγt + ILCs ( Fig. 5c ). Both RORγt + ILCs isolated from DOCK8 pri/pri or WT control mice had comparable level of expression of IL-7Rα. Thus, RORγt + ILC defects in DOCK8-deficient mice are not due to defective IL-7 expression ( Fig. 1f , right panel) in the gut or defects in IL-7Rα expression on these cells. Next, we explored whether DOCK8-deficient ILC3 had normal response to IL-7 stimulation. Thus we isolated cells from SI LPLs of Rag1 −/− IL-23R gfp/+ and Rag1 −/− IL-23R gfp/+ DOCK8 pri/pri mice and measured phosphorylation of STAT5 (pSTAT5) in response to IL-7. To our surprise, DOCK8-deficient ILC3s could not phosphorylate STAT5 as efficiently as WT ILC3s ( Fig. 5d ). DOCK8-deficient ILC3s have an impaired IL-7 mediated signalling, which may compromise their survival in the gut. All together, these data suggest that DOCK8 is critical for protective immunity against enteric pathogen by regulating the generation and survival of RORγt + ILCs in the GI tract. In the present study, we have described how a deficiency in DOCK8 leads to compromised protective immune response against an enteric pathogen. We have shown that DOCK8 expression in the haematopoietic compartment is required for protective immunity and its deficiency results in drastic reduction of RORγt + ILCs in the GI tract. We have also presented evidence that DOCK8 positively regulates the survival of RORγt + ILCs in a cell-intrinsic manner. The development of RORγt + ILCs is dependent on several transcription factors including Id2 (refs 4 , 50 ), RORγt [51] ,Tox [52] and Ikaros [55] . Our studies show that DOCK8 is not required for the development of fetal LTi cells because DOCK8-deficient mice, in contrast to RORγt-deficient mice, develop normal LNs and have normal LTi cells in their GI tract, so it is therefore likely that DOCK8 plays an important role in the maintenance of RORγt + ILCs after birth or in adult mice. Our findings have uncovered a previously unsuspected role for DOCK8 in protective immunity at GI tract mucosa. Recently, Ahr was shown to be important for the generation and maintenance of adult RORγt + ILCs [10] , [37] , [38] . More recently, the transcription factor T-bet (encoded by Tbx21 ) was also shown to be critical for the development of NKp46 + ILC3 (refs 56 , 57 , 58 ). However, neither Ahr nor T-bet is required for the generation of fetal lymphoid tissue inducer (LTi) cells and as a result, these mice have normal LN formation. Unlike the above-mentioned transcription factors, DOCK8 is unique in that it is not affecting a particular subset of ILC3, but is required for the survival of all RORγt + ILCs, including both CD4 + and NKp46 + subsets. The absence of DOCK8 may influence the microbial composition in the GI tract and that may influence the RORγt + ILCs generation or survival. However, it is still under debate whether the development of IL-22-producing ILCs requires intestinal symbiotic microbes [11] , [36] , [42] , [46] , [54] , [58] . Our mixed bone marrow chimeric experiment has further demonstrated that RORγt + ILCs from DOCK8-deficient mice are impaired in a cell-intrinsic manner. Although our findings indicate that DOCK8 is required for the generation and survival of RORγt + ILCs, DOCK8 is also important for the survival and function of CD8 + T cells [25] and NKT cells [35] . Therefore, DOCK8 in general may be required for the survival of many immune cells. However, more studies are required to determine by which mechanisms DOCK8 regulates cell survival. DOCK8-deficient patients develop atopic dermatitis, Staphylococcus aureus skin abscesses or soft tissue infections, pneumonias, elevated serum IgE, eosinophilia and GI tract infections [21] , [23] , [59] . The majority of these patients have low numbers of CD4 + and CD8 + T cells in the blood and spleen [21] . However, it has not been investigated whether DOCK8-deficient patients also have defects in ILCs or altered microbial composition in their GI tracts. It is critical because dysbiosis in the microbial community can result in inflammatory diseases not only of the intestine, but also of organs at distal sites [60] . It is widely accepted that RORγt + ILCs are critical for protective immunity at barrier surfaces [11] , [36] . Therefore, our findings that DOCK8 is required for the generation of RORγt + ILCs provides additional insight on the clinical features and the severe immunodeficiency observed in DOCK8-deficient patients. Recent data have provided evidence that commensal bacterial-derived signals limit steady-state serum IgE concentration and basophil-associated allergic inflammation [61] . Since DOCK8-deficient patients have an autosomal recessive form of hyperimmunoglobulinemia E syndrome characterized by recurrent infections, increased susceptibility to atopic eczema and average serum IgE concentrations 10 times higher than those found in control subjects [21] , [22] , it is tempting to speculate that the increased susceptibility to bacterial infection and the elevated levels of IgE seen in DOCK8-deficient patients could be the result of dysbiosis in the microbial community or inadequate control of pathogens due to a defect in the surveillance of the GI tract by ILCs. In addition to infection susceptibility, DOCK8-deficient patients also have higher susceptibility to cancer [21] , [23] , [59] . Using a mouse model, it has been shown that NKp46 + LTi cells are essential for melanoma rejection mediated by IL-12 (ref. 62 ). In the above study, authors showed that IL-12-mediated repression of subcutaneous melanoma is independent of adaptive immunity or cNK cells, but requires innate linease-negative NKp46 + LTi cells. Tumour rejection by NKp46 + LTi was independent of IFN-γ, IL-22, lymphotoxin, perforin or IL-17, but required the expression of adhesion molecules in tumour vessels, which could facilitate the ability of leukocytes to evade the tumour [62] . Thus, our findings that DOCK8-deficient mice have drastic reductions in RORγt + ILCs could explain why DOCK8-deficient patients are more prone to cancer. In summary, our data show that DOCK8 is critical for protective immunity against enteric pathogen infection, independent of its role in B-cell-mediated functions. Our findings have revealed an unanticipated DOCK8 requirement for the generation and survival of RORγt + ILCs. We also provide evidence that drastic reductions in the numbers of RORγt+ ILCs, as well as defective IL-22 production by these cells, are responsible for early mortality on C. rodentium infection in DOCK8-deficient mice. To our knowledge, this is the first study that has identified the scaffolding protein DOCK8 as an important molecule for the generation, survival and optimal function of ILCs and protective immunity against enteric pathogen. Given that DOCK8 deficiency in human patients results in recurrent infections and increased vulnerability to cancer, these consequences may partly be due to defective RORγt + ILCs in the GI tract. Mice Mice were bred and maintained under specific pathogen-free conditions in accordance with animal facilities at the Seattle Children’s Research Institute (SCRI). Experiments were conducted in accordance with the guidelines of the SCRI Animal Care and Use Committee. IL-23R −/− and DOCK8-deficient (DOCK8 pri/pri ) mice were generated as previously described [24] , [45] . WT (C57BL/6) and Rag1 −/− mice were purchased from Jackson Laboratories (Bar Harbour, ME), while Rag2 −/− IL-2Rγ −/− mice were purchased from Taconic. Most of the animals used in the study were 6–8-weeks old male and female mice. C. rodentium infection and assessment of CFU C. rodentium was cultured overnight at 37 °C in Luria broth with gentle agitation. After spinning down at 4,500 r.p.m., they were suspended in PBS and the concentration was measured using a 600 nm cell density metre (WPA Biowave CO8000). Mice were fasted for 8 h before oral gavage of 2 × 10 9 colony-forming units in 200 μl PBS. Spleens and livers of infected mice were used to analyse the colony-forming units. Spleens and livers were mechanically crushed in PBS and after serial dilution, plated on LB agar plates and incubated overnight at 37 °C. Bone marrow transfer Donor bone marrow cells (5 × 10 6 ) were intravenously injected into recipient mice irradiated at 550 rads. Irradiated mice were treated with antibiotics (Baytril) for 2 weeks after injection and mice were infected 6 weeks post transfer. Mixed bone marrow transfer Recipient Rag2 −/− IL-2Rγ −/− mice were irradiated 4 h before transfer at 550 rad and treated with antibiotics (Baytril) for 2 weeks. Irradiated mice received 50/50 mixture of CD45.1 + WT and CD45.2 DOCK8 pri/pri bone marrow cells (5 × 10 6 ) intravenously and mice were analysed for RORγt + ILCs 5 weeks post transfer. Isolation of LP cells For GI tract LPL isolation, colons and SI were isolated, flushed with ice-cold PBS, the attached fat removed and then cut open longitudinally. The samples were cleaned by shaking in ice-cold PBS four times before tissue was cut into 1 cm pieces. The epithelial cells were removed by incubating the tissue in predigestion buffer (HBSS, 2 mM EDTA and antibiotics) for 30 min at 37 °C with shaking. The LPL cells were isolated by incubating the tissues in digestion buffer (HBSS, 10% fetal bovine serum, 1 mg ml −1 Collagenase (Worthington) and DNase (Sigma-Aldrich) for 20 min. The digested tissues were then filtered through a 40-μm filter. This step was repeated to get the complete digestion of the tissues. Cells were washed once in the ice-cold medium (RPMI, 10% fetal bovine serum and antibiotics), resuspended in 10 ml of the 40% fraction of a 40:80 Percoll gradient and overlaid on 5 ml of the 80% fraction in a 15 ml Falcon tube. Percoll gradient separation was performed by centrifugation for 20 min at 1,800 r.p.m. at room temperature. LPL cells were collected at the interphase of the Percoll gradient, washed and resuspended in medium. Flow cytometric analysis For flow cytometric analysis, cells were stained with antibodies to the following markers: CD3 ((FITC or PE, eBioscience, alexa fluor 647, BioLegend) (1:250 dilution)), CD90.2 ((PE-Cy5, PE-Cy7 Biolegend; 1:2,000 dilution)), CD4 ((PE, PE-Cy5, APC-efluor 780 or efluor 450, eBioscience; 1:250 dilution)), IL-22 ((APC, eBioscience; 1:125 dilution )), RORγt ((PE, eBioscience; 1:200 dilution)), CD127 ((PE or APC-efluor 780, eBioscience), NKp46 (eflour 660, eBiosciences), c-Kit (PE-Cy7, BD Biosciences; 1:125 dilution)), SCA-1 ((PerCP-Cy5.5, eBiosciences; 1:500 dilution)), CD8 ((PE-Cy7, eBioscience; 1:2,500 dilution)), CD19 ((FITC, eBioscience), B220 (Alexafluor 647, Biolegend; 1:500 dilution)), MHC class II ((PE, eBioscience), CD11c (APC, eBioscience) and CD11b (APC-efluor 780, eBioscience; 1:500 dilution)). For cytokine production, cells were stimulated directly ex vivo by incubating for 4 h with 20 ng ml −1 IL-23 (eBioscience) in the presence of Golgi plug (BD). Cells were fixed and permeabilized by using Foxp3 fix/perm buffer set Cat# 421403 (Biolegend), as described by manufacturers and stained with IL-22 and RORγt. For pSTAT3, cells were stimulated by incubating for 20 min with 50 ng ml −1 rIL-23 (eBioscience) followed by fixation with 2% paraformaldehyde. Paraformaldehyde-fixed cells were permeabilized with phosflow perm buffer III (BD biosciences) and stained with anti-STAT3 (pY705) antibody conjugated to Alexa fluor 647 (BD biosciences). Gene expression Total RNA was extracted with Trizol (Invitrogen, Carlsbad, CA) and reverse transcribed with the iScript cDNA synthesis kit (BioRad, Hercules, CA). The real time PCR was conducted using Step One Plus Real Time PCR system (Applied Biosystems) with primer and probe listed in Supplementary Table 1 . The reaction was set using Taq Man Fast Universal PCR Master Mix Cat# 43552042 (Applied Biosystems). The samples were normalized to the control housekeeping gene RPL-19 and reported according to the dC T method. Measurement of IL-22 by ELISA Sorted SI LPLs (3,000) were cultured in the absence or presence of 20 ng ml −1 rIL-23 (eBioscience CA, USA) for 24 h. The supernatant was centrifuged and measured for IL-22 protein concentration by sandwich ELISA kit #88-7522-86 (eBioscience CA, USA). Hydrodynamic gene delivery of IL-22 For hydrodynamic injections, 15 μg plasmid DNA was resuspended in 2 ml of PBS and intravenously injected in 5–10 s using hydrodynamic tail vein injection. IL-22 protein production was validated from blood of mice that had received the hydrodynamic plasmid injections. RNA sequencing Total RNA was purified from C. rodentium infected colon with RNeasy mini kit (Qiagen). RNA sequencing was performed at Genomic Core Facility Southwestern Medical Center, University of Texas. Statistical analysis For statistical analysis, P values were calculated with a two-tailed unpaired Student’s t -test. P values of less than 0.05 were considered significant. Error bars denote±s.d. How to cite this article: Singh, A. K. et al . DOCK8 regulates protective immunity by controlling the function and survival of RORγt + ILCs. Nat. Commun. 5:4603 doi: 10.1038/ncomms5603 (2014). Accession codes: RNA-sequencing data have been deposited in the gene expression omnibus (GEO) database under accession code GSE58765 .